Axis-dependence of molecular high harmonic emission in three dimensions High-order harmonic generation in an atomic or molecular gas is a promising source of sub-femtosecond vacuum ultraviolet coherent radiation for transient scattering, absorption, metrology and imaging applications. High harmonic spectra are sensitive to Ångstrom-scale structure and motion of laser-driven molecules, but interference from radiation produced by random molecular orientations obscures this in all but the simplest cases, such as linear molecules. Here we show how to extract full body-frame high harmonic generation information for molecules with more complicated geometries by utilizing the methods of coherent transient rotational spectroscopy. To demonstrate this approach, we obtain the relative strength of harmonic emission along the three principal axes in the asymmetric-top sulphur dioxide. This greatly simplifies the analysis task of high harmonic spectroscopy and extends its usefulness to more complex molecules. Over the last two decades, high harmonic generation (HHG) has emerged as an important technique to explore both electron structure [1] and sub-femtosecond dynamics [2] , [3] . HHG sources using rare gases have become workhorses for general vacuum ultraviolet spectroscopy and anticipate a new generation of precision measurement tools [4] , [5] . A better understanding of high harmonic processes will likely lead to new applications in chemical physics involving molecular bonds, and in the attosecond physics of electrons in molecules. HHG target gases of linear molecules such as molecular nitrogen (N 2 ) or carbon dioxide (CO 2 ) can be prepared with a preliminary laser impulse that transiently aligns the molecules in advance of the more intense harmonic generation pulse [6] . The high sensitivity of HHG to the shape and binding energies of molecular orbitals gives the system a rich angle-dependent harmonic spectrum. HHG from aligned molecules can help test strong-field theories of harmonic generation and reveal complex effects such as contributions from multiple orbitals [7] , [8] , [9] or from the shape of a single molecular orbital [3] , [10] , [11] as long as the system can be interpreted in the molecular frame. However, polyatomic molecules generally have multiple moments of inertia and a complicated polarizability tensor so they cannot be aligned in the laboratory frame by a simple stimulated Raman pulse. In general, molecular axes are not aligned with the laser polarization direction at a given point in time. Thus, for a three-dimensional molecule, the radiated field arising from the molecule may have a different nonzero component along each molecular axis. The question of whether the HHG signal gets stronger or weaker or even changes its phase as well as magnitude, when the angle between an axis and the laser polarization varies, is answered by our analysis. The molecule is not a different molecule when it rotates a few degrees. However, the response of the molecule to a driving field may indeed depend on this angle. The coherent superpositions of the harmonic fields from different randomly oriented molecules in the molecular ensemble complicate the conversion from the laboratory frame into the more useful molecular frame. This is the information that our analysis can extract. Here, we show how body-centered angle-dependent information can be obtained from complex three-dimensional target molecules in gas phase by an approach that is conceptually similar to rotational coherence spectroscopy [12] . This method has been used to determine the rotational constants and the polarizability tensor of asymmetric-top molecules. We use it to analyse high harmonic data. This allows us to obtain the molecular-frame axis-dependent amplitude and phase of harmonic emission. Three-dimensional molecular rotations A three-dimensional, asymmetric-top molecule undergoes periodic transient alignments along each of its three inertial directions as different quantized orbitals come into phase. There can be up to five different types of these quantum rotational wavepacket quasi-revivals following a single kick, which form a unique molecular fingerprint (see Supplementary Note 1 ). Each molecular axis has a unique pattern of quasi-revivals following the impulse that created the rotational coherences. These single-axis, quasi-revival patterns are basis functions on that time axis. We project the HHG signal onto these functions to decompose it. As depicted in Fig. 1 , this procedure allows us to convert our signal into the molecular frame by reconstructing the components along each molecular axis. This yields complex coefficients that reveal the relative amplitude and phase of harmonic emission from each axis. 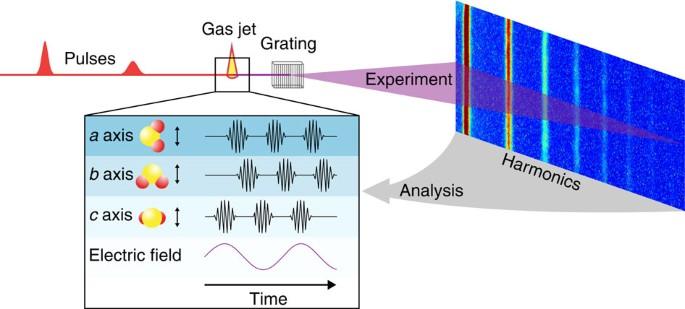Figure 1: The alignment decomposition approach. We make use of an initial kick to molecules in a gas to create a rotational coherence. A second pulse generates high harmonics to probe the molecule, which can be viewed using a grating spectrometer. For simpler symmetric-top molecules, the kick leads to periodic alignment, so harmonics generated at the times of greatest alignment can be related to the molecular frame of the molecule. But in an asymmetric top, as considered here, there is no simple correspondence between coherent transient features and alignment of any single axis in the molecule. No axis has a single characteristic time constant for periodic quantum revivals; rather, each axis has a unique temporal pattern of alignment following the kick. Since these patterns of molecular alignment along each molecular axis are unique, we can decompose the HHG emission pattern (top), projecting out the contributions from each molecular axis. To decompose the HHG signal, we fit single-axis alignment patterns to our data to obtain the amplitude and phase from each molecular axis (bottom). The single-axis alignment patterns are the expectation values of molecular alignment along each axis that serve as basis vectors for our fit. Figure 1: The alignment decomposition approach. We make use of an initial kick to molecules in a gas to create a rotational coherence. A second pulse generates high harmonics to probe the molecule, which can be viewed using a grating spectrometer. For simpler symmetric-top molecules, the kick leads to periodic alignment, so harmonics generated at the times of greatest alignment can be related to the molecular frame of the molecule. But in an asymmetric top, as considered here, there is no simple correspondence between coherent transient features and alignment of any single axis in the molecule. No axis has a single characteristic time constant for periodic quantum revivals; rather, each axis has a unique temporal pattern of alignment following the kick. Since these patterns of molecular alignment along each molecular axis are unique, we can decompose the HHG emission pattern (top), projecting out the contributions from each molecular axis. To decompose the HHG signal, we fit single-axis alignment patterns to our data to obtain the amplitude and phase from each molecular axis (bottom). The single-axis alignment patterns are the expectation values of molecular alignment along each axis that serve as basis vectors for our fit. Full size image Our results show that HHG is a powerful tool to probe increasingly complex molecules. Our approach is generalizable to any molecule that can exhibit quantized rotational coherences and to techniques beyond HHG. Most molecules are asymmetric tops and even reactions with linear molecules generally proceed via an asymmetric-top transition state. Thus, an alignment decomposition into three dimensions is a solution that could be employed by much of the ultrafast molecular science community, enhancing or augmenting techniques such as time-resolved X-ray [13] , [14] and electron diffraction [15] , [16] , photoelectron spectroscopy [17] , [18] , as well as HHG [19] , [20] . As a test case for our approach we chose to analyse the HHG production along each of the principal axes of the asymmetric-top molecule sulphur dioxide (SO 2 ). This molecule has many compelling features, such as several molecular orbitals with different symmetries within a few eV of the highest occupied orbital (HOMO). It also has several unoccupied excited bound states that have been proposed for HHG studies of intramolecular dynamics [21] . Our experimental scheme employs two pulses with parallel polarizations: one to deliver the impulse to the molecular gas and one to produce HHG from the resulting rotational coherent states. We vary the time delay between the two pulses to record the variations of HHG during transient coherent rotations induced by the first pulse. The HHG signal varies with this time delay, and this time variation can be decomposed into components corresponding to each alignment axis. Our experimental signal is shown in Fig. 2a . We observe a complex pattern of fractional revivals and multiple revivals of rotational wavepackets, with a revival sensitivity comparable to that seen in linear molecules in previous work [22] . This single pattern, which represents the 19th harmonic, contains evidence for all types of prolate-type asymmetric-top rotational revivals. A complete set of asymmetric-top revivals has not previously been recorded together in one trace. This shows the extreme sensitivity of HHG to small features in the alignment distribution (see Supplementary Tables 1 and 2 ). 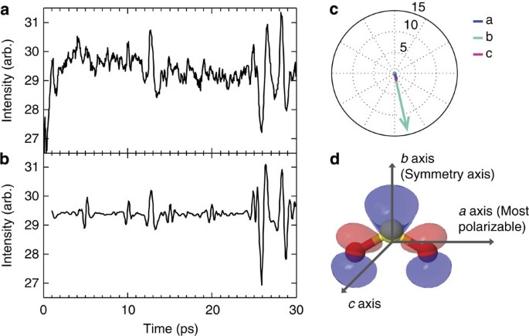Figure 2: Comparison between experiment and a best-fit theory curve. (a) Data for high harmonic 19 (29.5 eV) for the first 30 ps following alignment. The high harmonic data are very sensitive to SO2revivals. All prolate-type asymmetric-top revivals can be seen, including partial revivals and multiple revivals all on one curve. Partial revivals of order up to 1/16 revivals are visible. (b) The best-fit theory curve fits all three single-axis alignment patterns to the data. The fit coefficients yield the orientational information corresponding to the high harmonic emission along each of the three molecular axes. (c) A phasor plot representing the magnitude and direction of HHG emission as calculated by the best-fit curve. For this harmonic, emission from thebaxis dominates and the phase is similar for all axes. (d) An isosurface representation of the HOMO of SO2, shown in red and blue to encode the phase, is overlaid on top of a ball and stick model. We see the highest electron density in theb-axis direction, which should result in higher rates of ionization and recombination in this direction, in confirmation of our analysis. Figure 2: Comparison between experiment and a best-fit theory curve. ( a ) Data for high harmonic 19 (29.5 eV) for the first 30 ps following alignment. The high harmonic data are very sensitive to SO 2 revivals. All prolate-type asymmetric-top revivals can be seen, including partial revivals and multiple revivals all on one curve. Partial revivals of order up to 1/16 revivals are visible. ( b ) The best-fit theory curve fits all three single-axis alignment patterns to the data. The fit coefficients yield the orientational information corresponding to the high harmonic emission along each of the three molecular axes. ( c ) A phasor plot representing the magnitude and direction of HHG emission as calculated by the best-fit curve. For this harmonic, emission from the b axis dominates and the phase is similar for all axes. ( d ) An isosurface representation of the HOMO of SO 2 , shown in red and blue to encode the phase, is overlaid on top of a ball and stick model. We see the highest electron density in the b -axis direction, which should result in higher rates of ionization and recombination in this direction, in confirmation of our analysis. Full size image A few significant structures are immediately apparent in Fig. 2a : there is an initial alignment peak immediately following the impulse with a duration of less than 1 ps. A revival peak appears around 13 ps and a large and complex triple-peaked revival structure appears around 26 ps. These peaks, in addition to smaller ones, serve as distinguishing marks of the spectrum that we can use to decompose the signal into individual molecular axis contributions. Three single-axis alignment patterns, depicted in Fig. 3 , show the molecular alignment as viewed from each axis of the molecule. Single-axis alignment patterns are the usual measure of alignment, which is the expectation value <cos 2 θ j > in the rotational wavepacket. Here θ j is the angle between the polarization direction of the laser and the molecular axis j . The molecular alignment is calculated with respect to all three molecular axes, a , b and c , which are defined in Fig. 3h . Although in this experiment we use HHG as the probe, the single-axis alignment patterns are not dependent on the particular alignment detection scheme used. The alignment patterns together represent ideal alignment. 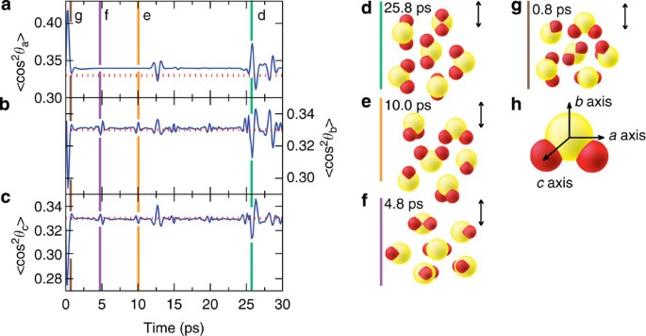Figure 3: Single-axis alignment patterns and molecular distributions. (a–c) Expectation values of alignment between molecular directionsa–cand the polarization direction of the HHG-probing pulse. For an isotropic distribution of molecular axes, <cos2θ>=1/3. (d–g) Idealized sample distributions at different revival times. The laser polarization direction is indicated. Note that there is no one-to-one correspondence between a particular axis and a revival type. Revivals must be read by considering all three single-axis alignment patterns simultaneously. A peak in a given curve indicates preferential alignment along the corresponding axis. (d–f) Alignments along axesa,bandc, respectively. (g) An isotropic distribution. (h) Molecular axes for SO2. Figure 3: Single-axis alignment patterns and molecular distributions. ( a – c ) Expectation values of alignment between molecular directions a – c and the polarization direction of the HHG-probing pulse. For an isotropic distribution of molecular axes, <cos 2 θ >=1/3. ( d – g ) Idealized sample distributions at different revival times. The laser polarization direction is indicated. Note that there is no one-to-one correspondence between a particular axis and a revival type. Revivals must be read by considering all three single-axis alignment patterns simultaneously. A peak in a given curve indicates preferential alignment along the corresponding axis. ( d – f ) Alignments along axes a , b and c , respectively. ( g ) An isotropic distribution. ( h ) Molecular axes for SO 2 . Full size image Extraction of electric field contributions For asymmetric tops, the signal will contain coherent contributions corresponding to the radiated electric field components along each of the molecular axes. The particular amount of each component is determined by the instantaneous molecular alignment, which is given by the three single-axis alignment patterns considered in tandem. We can thus use the single-axis alignment patterns as basis vectors, f j , along which the data are decomposed. It is important to note that we do not model the probe signal by alignment; rather, we extract the particular molecular alignment that caused the probe signal. Determining the relative orientation of the molecular axes to the laboratory polarization axis yields a rotation matrix that allows us to project the probe signal back into the molecular frame. In such a way we can obtain the HHG emission along all three molecular-frame directions without resorting to modelling the harmonics. Since electric field contributions with the same polarization add coherently, we allow for an amplitude, c j =| c j |, and a phase, θ j , for the component of the probe electric field arising from each molecular direction j . Physically, the three coefficients c j =| c j | are none other than the components of the radiated electric field in the molecular frame. These are then summed and squared according to the form F j = to obtain an intensity that is comparable to an experimental signal. To determine the numerical value of the coefficients for a particular time-delayed harmonic scan, we use the amplitudes and phases as fit parameters to match the combined alignment patterns to the data. To extract the parameters, we minimize χ 2 according to the usual formula for χ 2 , , where d corresponds to our data, to obtain the best possible fit using a Nelder–Mead fitting procedure [23] (see Supplementary Discussion ). This allows us to extract separately the amplitudes and phase that most accurately represent the high harmonic emission of our data. In the absence of external phase information, only the relative phase of the three coefficients is meaningful. The phase information may be particularly useful because it suggests the underlying HHG processes of field emission and recombination [20] . The results are shown in Fig. 2b . The extracted fit coefficients for the magnitude of the electric field are for axes a : b : c on an arbitrary scale. For the phase the fit coefficients are radians. The χ 2 for the fit is 0.56 with 120 d.f. (see Supplementary Table 3 ). The fit coefficients are shown in a phasor diagram in Fig. 2c . We conclude that for this harmonic emission the dominant contribution to HHG emission comes primarily from molecules aligned with the C 2v ( b ) axis along the polarization direction. There is some emission along the a and c directions as well, but their magnitude is small compared with the b axis. Moreover, the phase is approximately the same for all three axes, so the b axis retains its effective dominance even after interference. Our data further indicate that harmonic emission is suppressed at orientations along the a axis, where the polarizability is largest. The high contribution to harmonic emission from the b axis could be due to either enhanced field ionization or enhanced recombination along this axis, according to the standard recollision model [24] , [25] , [26] . To provide a check for the method, we model the energy- and angle-dependent recombination dipole by calculating the VUV photoemission cross-section of SO 2 in the molecular frame, as shown in Fig. 4 . 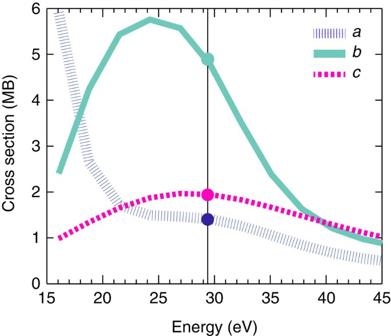Figure 4: Recombination cross-section of SO2. The cross-section is plotted as a function of photon energy. The laser polarization is oriented along thea-,b- andc-axes of the molecule in the dotted blue, solid green and dashed red curves, respectively. High harmonic 19 has ~29.5 eV of energy; at this point the recombination cross-section is much higher along the molecular symmetry axis (baxis) than along either of the other two axes. This indicates that there is higher recombination probability along thebaxis than along the other two axes and provides another confirmation of the validity of our approach. Figure 4: Recombination cross-section of SO 2 . The cross-section is plotted as a function of photon energy. The laser polarization is oriented along the a -, b - and c -axes of the molecule in the dotted blue, solid green and dashed red curves, respectively. High harmonic 19 has ~29.5 eV of energy; at this point the recombination cross-section is much higher along the molecular symmetry axis ( b axis) than along either of the other two axes. This indicates that there is higher recombination probability along the b axis than along the other two axes and provides another confirmation of the validity of our approach. Full size image We find that recombination is a major contribution to the magnitude of harmonic emission along different molecular axes. At our signal energy of 29.5 eV there is a large recombination probability along the molecular symmetry axis, but much less recombination along the other two axes. This is consistent with the results of our fit, and helps to validate the fitting procedure. We compared our results from the HOMO with other valence orbitals (see Supplementary Information ). The recombination dipole dependence on geometry for these orbitals suggests that our signal arises primarily from the HOMO. This is consistent with results for low harmonics in other molecules [7] , [9] . As a second check for the fit, we can examine the orbital structure for SO 2 shown in Fig. 2d . Since there is greater electron density along the symmetry axis there is a higher recombination probability in that direction than along the other two directions, even than along the most polarizable axis direction. The method we have presented here thus provides a way to decompose the HHG emission amplitude and phase along each principal axis of an asymmetric top. This information is crucial for understanding the strong-field response of asymmetric-top molecules. An advantage of this method is that it uses only a single impulse to extract information about all three molecular axes. It removes the necessity to align a polyatomic molecule along all three dimensions, an onerous requirement that places a burden on the amount of laser power needed. We expect that alignment decomposition will be useful for studies of angle-dependent molecular structure and dynamics as well. We make three assumptions in carrying out this approach. This first is that the principal of superposition holds; this holds true here, as it does for all identically polarized electric fields. The second is that molecular alignment is well modelled by <cos 2 θ >. While this is the usual assumption, it presumes molecular rigid rotors and may not hold for molecules with a rotational Raman cross-section small compared with internal modes. The third assumption is that the asymmetric-top molecular coherences are experimentally visible. This approach is completely generalizable if the above assumptions are fulfilled. In this simple example case, the HOMO orbital of SO 2 has its maximal values along the principal axes of the molecule. Thus, it was sufficient to use only parallel polarizations between the pump and probe pulses to extract these values. However, we might repeat the same approach along any polarization angle with respect to the driving field. This would allow us to obtain enough information to undertake a full reconstruction. In such a way, this method would be useful for molecules that have their maximal value at angles not along the principal molecular axes as well. Several researchers have attempted a full tomographic reconstruction from the angle-dependent HHG in aligned linear molecules [1] , [27] , [28] . It would be very interesting to collect a full angular map of HHG in an asymmetric top, because we expect HHG to have a complicated relationship to molecular structure owing to its dependence on strong-field tunnelling and quantum orbital interference. Moreover, the ability to observe revivals in asymmetric tops with precision up to the 1/16 revival confirms the HHG sensitivity seen by Lock et al . [22] , and offers an interesting system for quantum control studies. Since five different prolate-type asymmetric-top revivals are visible in the data, quantum control techniques could be employed to enhance or, alternatively, suppress any particular revival. For example, by repetitively pulsing [29] at interval times corresponding to each of the three rotational periods of the molecule, alignment traces correlated to each axis’s revivals ought to become visible. The evolution across different harmonics might reveal attosecond dynamics corresponding to a particular molecular rotation [30] . Alternatively, by varying laser intensity or wavelength, a phase shift in emission might become observable using this technique, indicating electron wavepacket motion. Analysing the harmonic signal We use impulsive-stimulated rotational Raman scattering to excite rotational coherences in a sample of SO 2 molecules. Following the impulse, the SO 2 is free to rotate, exhibiting a quasi-revival structure that is determined by the field-free rotational spectrum. We probe the SO 2 at various time delays by using a focused 30 fs pulse with a central wavelength of about 780 nm, a pulse energy of about 53 μJ, a repetition rate of 1 kHz and a focusing lens with f=150 mm to produce HHG in the SO 2 gas. The coherent impulse is constructed from the same laser, but the pulses are temporally dispersed to a pulse duration of 130 fs using 16 mm of BK7 glass. The impulse has a pulse energy of ~28 μJ. The HHG pulse follows the alignment pulse through the gas jet in a collinear fashion. Both laser beams are linearly polarized. Harmonics produced in jet and between 25 and 55 eV pass through an aluminium filter with a thickness of 100 nm onto a spherical grating. The time delay between the impulse and HHG generation pulse is incremented in steps of 47.8 fs. Each 30 ps scan takes about 1.5 h to obtain a signal-to-noise ratio >25. The HHG is dispersed through a flat-field diffraction grating spectrometer and amplified with a bare microchannel plate and detected on a phosphor screen. This is then recorded using a charge-coupled device camera. The molecules are introduced through an expansion nozzle located above the laser focus and thus collisionally cooled (see below). The HHG signal is affected by the grating acceptance, as well as by phase matching and volume averaging effects. However, none of these impacts the information that we need to extract from the fit. The phase matching is almost completely determined by geometry and remains constant throughout the time delay scan. The signal also contains contributions from different impulse strengths across the laser focus. But again, this volume imaging affects all time delays equally and therefore does not obscure our signal. We chose harmonic 19 for this study, because we wanted to concentrate on a harmonic that was intense and thus more immune to statistical noise, but at the same time also in the high-harmonic plateau region and far from the cutoff, where the results are strongly dependent on intensity. We also wanted a harmonic that would be far from the lower order harmonics, where the standard three-step model is less valid. We estimate the temperature by assuming a supersonic expansion. We calculate the backing density, 2.43 × 10 19 cm −3 , by using the equation of state for an ideal gas with a backing pressure of 1 bar and room temperature. Our uncertainty stems mainly from our lack of precise knowledge of how far exactly the high harmonic jet is from the laser focus, x, and precisely how large our tip diameter, d , is. Our best estimate for this parameter is 0.033< <1. In Scoles et al . [31] , the authors show that for a supersonic gas jet, where T 0 represents the initial temperature, T represents the final temperature, γ is the heat capacity ratio (1.29 for SO 2 ) and M is the Mach number for the supersonic expansion. M is calculated by Scoles et al . [31] The authors show that for a supersonic gas jet, for 0< <1. A and B are the Mach number correlation parameters for axisymmetric expansion and are given by A=3.61 and B=1.95. From these equations we are able to estimate the temperature of the gas jet at the laser focus as 240±20 K. Theory of single-axis alignment patterns Our theory and numerical approach for solving the time-dependent Schrödinger equation of an asymmetric-top molecule interacting with an aligning field is based on the theory of stimulated Raman scattering [32] , [33] . In brief, for the duration of the laser pulse, the rotational wavefunction is expanded in a symmetric top basis, | JKM , thus converting the time-dependent Schrödinger equation into a set of coupled differential equations that are solved numerically. Here J , K and M denote the quantum numbers corresponding to the total angular momentum and its projections onto the body- and space-fixed z axes. Note that K is not a conserved quantum number for an asymmetric top. The pulse is modelled as a Gaussian. After the pulse turn-off, the wavefunction is transformed to the basis of eigenstates of the field-free Hamiltonian. The principal components of the polarizability tensor were determined in ref. 34 . The total Hamiltonian is H ( t )= H rot + H ind ( t ). The rotational Hamiltonian in the rigid-rotor approximation is H rot = , where B K and J K , k = X , Y, Z, are the rotational constant components of the angular momentum operator, respectively. The body-fixed frame is defined by setting the X , Y and Z axes parallel to the molecular c , b and a axes. In the space-fixed frame, the laser field polarization vector defines the z axis. The field–matter interaction Hamiltonian is where ɛ ( t ) is the aligning pulse Gaussian envelope, are Wigner rotation matrices [35] , and α kk ′ = α kk − α k ′ k ′ are the generalized polarizability anisotropies with α kk being the body-fixed frame components of the polarizability tensor taken from ref. 34 . The aligning pulse duration and intensity in the calculation are taken to be the same as used in our experiments. The rotational wavefunction is expanded in a symmetric top basis, | JKM , Here J , K and M denote the quantum numbers corresponding to the total angular momentum and its projections onto the body- and space-fixed z axes. The matrix elements of H rot in this basis are easily evaluated analytically [35] . Likewise, the matrix elements of H int are analytical and given as superpositions of integrals of the form H rot conserves the M quantum number. The K quantum number is not conserved here, but because of the cylindrical symmetry of the linearly polarized field, M is also conserved by H ind . Because M remains a good quantum number, the wavefunction is effectively two-dimensional with only parametric dependence on M , that is, The time-dependent Schrödinger equation is thus converted into a set of coupled differential equations to be solved numerically, that is, After the pulse turn-off, when the envelope tail is truncated as it becomes sufficiently small, the wavefunction is transformed to the basis of eigenstates of the field-free Hamiltonian, H rot . The alignment observables are cos 2 θ i , i = a , b , c , where θ i is the angle between the laser field polarization direction and molecular axis i , The observables are calculated for a thermal ensemble, where the sum runs over all thermally populated initial states, ( t ) is a state-specific observable, and ω i ( T ) are normalized weight functions consisting of the Boltzmann factor and nuclear spin statistical weight [36] . The aligning pulse duration and intensity in the calculation are taken to be the same as used in our experiments. The observables are calculated for a thermal ensemble corresponding to the temperature of 180 K, the highest temperature that was computationally feasible. Since the method relies on the position of revival features and revival position is independent of temperature, this discrepancy between the temperature of the experiment and the calculation only has a minor effect on the fitting procedure. Computation of recombination cross-sections We compute fixed-nuclei photoionization amplitudes using the complex Kohn variational method [37] . This gives us information about the recombination physics, because the recombination step in HHG is equivalent to inverse photoionization. Here we give a brief summary. The final-state electronic wavefunction for production of photoions is in a specific cation state Γ 0 with an initial angular momentum l 0 m 0 is written as where Γ labels the ionic target states χ Γ included and F are channel functions that describe the incoming electron, A is the antisymmetrization operator and the Θ i s are N electron correlation terms. In the present application, only one ionic target state, the 8a 1 −1 hole state, was included in the trial wave function. In the Kohn method, the channel functions are further expanded, in the molecular frame, as where the ϕ i ( r ) are a set of square-integrable (Cartesian Gaussian) functions, Y lm is a normalized spherical harmonic, k Γ are channel momenta and the f lm ( k Γ , r ) and ( k Γ , r ) are numerical continuum functions that behave asymptotically as regular and outgoing partial-wave Coulomb function, respectively [38] . The coefficients are the T-matrix elements. Photorecombination cross-sections in the molecular frame can be constructed from the matrix elements where r μ is a component of the dipole operator, which we evaluate here in the length form, and Ψ 0 is the initial-state wavefunction of the neutral N electron molecule. Ψ Γ 0 l 0 m 0 is the cation ground state with a continuum electron described by the quantum numbers. In order to construct an amplitude that represents an electron with momentum recombining with the molecule and ejecting a photon with polarization direction , measured relative to the molecular body-frame, the matrix elements must be combined in a partial wave series where is a Coulomb phase shift. The cross-section, differential in the angle of incoming electron and photon polarization relative to the fixed body-frame of the molecule, is then given by where ω is the photon energy and c is the speed of light. Finally the cross-section for a particular polarization direction μ is given by Further details can be found elsewhere [39] , [40] . To ensure that our signal was arising only from the HOMO of SO 2 and not lower-lying orbitals, we compared the recombination dipole dependence for the HOMO-1 through HOMO-5. The ionization potentials for sulphur dioxide are 12.35 (HOMO, 8a 1 ), 12.99 (1a 2 ), 13.22 (5b 2 ), 15.90 (4b 2 ), 16.34 (7a 1 ) and 16.45 (2b 1 ) [41] . It is thus feasible that we might see some signal from several of the lower-lying orbitals, which are relatively close to the HOMO in energy. To determine whether this is the case, we consider molecular symmetries. The SO 2 molecule belongs to the C 2v point group. This group contains four irreducible representations: A 1 , A 2 , B 1 and B 2 . Each molecular orbital obeys the symmetries of one of these irreducible representations. On the basis of symmetries present in the group character table, we can assign nodal planes to the molecular orbitals of each of these four types. Since high harmonics are most likely to be ionized and recombined from directions with high electron density, a nodal plane implies minimal signal in that direction. Our analysis shows a strong signal from the b axis. Thus, the signal cannot arise from A 2 -, B 1 - or B 2 -type orbitals, which all have nodes along the b axes. The signal must be coming from an A 1 state. The only two orbitals that could thus potentially contribute are the HOMO (8a 1 ) and the 7a 1 orbital. The structure of the 7a 1 orbital contains only a very small lobe of electron density in the b axis direction and thus contributes very little to the total harmonic signal. These intuitions are corroborated by recombination cross-section calculations, which show that the HOMO orbital is the main contribution to the total signal. This analysis yields two important conclusions. First, for SO 2 , the C 2v symmetry implies that it is sufficient to investigate only a few directions to see which orbitals are responsible for the signal. In general we may need a full data set probing many different pump-probe angles to determine the orbital origin of the signal, but here this is sufficient. Second, the method is extendable to other molecules by making use of their symmetries in a comparable way. How to cite this article: Spector, L. S. et al . Axis-dependence of molecular high harmonic emission in three dimensions. Nat. Commun. 5:3190 doi: 10.1038/ncomms4190 (2014).